Fucose-based PAMPs prime dendritic cells for follicular T helper cell polarization via DC-SIGN-dependent IL-27 production Dendritic cells (DCs) orchestrate antibody-mediated responses to combat extracellular pathogens including parasites by initiating T helper cell differentiation. Here we demonstrate that carbohydrate-specific signalling by DC-SIGN drives follicular T helper cell (T FH ) differentiation via IL-27 expression. Fucose, but not mannose, engagement of DC-SIGN results in activation of IKKε, which collaborates with type I IFNR signalling to induce formation and activation of transcription factor ISGF3. Notably, ISGF3 induces expression of IL-27 subunit p28, and subsequent IL-27 secreted by DC-SIGN-primed DCs is pivotal for the induction of Bcl-6 + CXCR5 + PD-1 hi Foxp1 lo T FH cells, IL-21 secretion by T FH cells and T-cell-dependent IgG production by B cells. Thus, we have identified an essential role for DC-SIGN-induced ISGF3 by fucose-based PAMPs in driving IL-27 and subsequent T FH polarization, which might be harnessed for vaccination design. Antibody-mediated responses are crucial to combat extracellular pathogens [1] . Humoural immunity is mediated by both type 2 T helper (T H 2) cells and follicular T helper (T FH ) cells that provide cognate help to B cells [2] . Establishment of protective long-term humoural immunity against extracellular pathogens such as parasites depends on the generation of high-affinity antibodies, a process that relies on formation of follicular structures called germinal centres (GCs) during infection. T FH cells form a specialized subset of effector CD4 + T cells required for GC formation. Once formed, T FH cells maintain GCs and regulate the differentiation of GC B cells into memory B cells and long-lived plasma cells. T FH cells produce interleukin (IL)-21, a potent cytokine that drives antibody isotype class switch recombination and B-cell proliferation, together with other factors [2] , [3] . Once B cells are outside GCs, IL-4 produced by T H 2 cells induces isotype switching to immunoglobulin E (IgE) antibodies [4] , [5] , [6] , which are integral in eosinophil-mediated killing and expulsion of parasitic worms from the intestines [1] , [7] . Sequential switching of IgG cells to IgE is essential for the development of long-lived high-affinity IgE + plasma cells [8] . T helper cell (T H ) differentiation is under the control of dendritic cells (DCs) that sense invading pathogens through pattern recognition receptors, which triggers innate signalling that drives T H polarization [9] , [10] . The factors involved in T FH polarization, including the role of DCs, are not clear. Initial T FH generation is thought to be driven by DCs, whereas B cells provide signals that reinforce the T FH phenotype and/or promote their survival [3] , [11] . IL-6 and IL-21 have important roles in vivo in the generation and maintenance of T FH cells and GC formation in mice, although conflicting data exist on their importance and redundancy in instructing T FH differentiation [12] , [13] , [14] , [15] , [16] , [17] , [18] . Since IL-21 is produced by activated T cells, it was proposed that IL-6 produced by DCs initially induces expression of transcription factor Bcl-6 (refs 13 , 15 ), which acts as the master regulator of T FH differentiation, including induction of IL-21 and chemokine receptor CXCR5, which is important for T FH homing to B-cell zones and GC formation [2] , [14] . Data on the requirements for human T FH differentiation are even more limited. We have previously shown that triggering of dendritic cell-specific intercellular adhesion molecule-3-grabbing non-integrin (DC-SIGN), a pattern recognition receptor from the family of C-type lectin receptors, modulates T H differentiation in a carbohydrate-specific manner [19] , [20] . The cytoplasmic tail of DC-SIGN is constitutively attached to adaptor protein LSP1 and the CNK-KSR1-Raf-1 signalosome, which are involved in downstream signalling when mannose-carrying ligands are recognized by DC-SIGN, leading to enhanced production of proinflammatory cytokines and T H 1 responses [19] . In contrast, priming of DCs by fucose-based glycan pathogen-associated molecular patterns (PAMPs) results in T H 2 differentiation [20] . Fucose-specific DC-SIGN signalling depends on crosstalk with Toll-like receptor (TLR) signalling and leads to activation of kinase IKKε in a LSP1-dependent but CNK-KSR1-Raf-1-independent manner. Subsequently, deactivation of deubiquitinase CYLD by IKKε-mediated phosphorylation leads to accumulation of ubiquitinated Bcl3 within the nucleus, where it modulates cytokine and chemokine expression by activated DCs to drive T H 2 polarization [20] . It is unknown whether DC-SIGN triggering also primes DCs for T FH polarization. Here we demonstrate that DC-SIGN triggering by fucose as well as fucose-carrying PAMPs from parasitic pathogens induces a specific innate signalling pathway that directs differentiation of T cells into Bcl-6 + CXCR5 + PD-1 hi Foxp1 lo T FH cells by DCs via IFN-stimulated gene factor 3 (ISGF3)-induced IL-27 expression. Fucose-specific DC-SIGN signalling activates kinase IKKε and crosstalk between IKKε and interferon-α/β receptor (IFNR) signalling—which is activated as a result of TLR-induced type I IFN synthesis—and promotes assembly of ISGF3, a multimeric transcriptional activation complex composed of STAT1, STAT2 and IRF9. ISGF3 positively regulates expression of IL-27 subunit IL-27p28 via recruitment of RNA polymerase II (RNAP2), enhancing the IL-27 transcription rate. DC-SIGN-dependent upregulation of IL-27 expression by DCs is crucial to the induction of Bcl-6 + T FH cells that secrete IL-21 and functionally induce IgG production by B cells. Thus, our data reveal an important role for DC-SIGN-IKKε signalling via crosstalk with IFNR signalling in priming DCs for T FH polarization. Furthermore, we have identified IL-27 as important for human T FH generation and the induction of humoural immunity to fucose-carrying extracellular parasitic pathogens. Fucose-specific DC-SIGN signalling leads to T FH polarization We investigated whether fucose-specific DC-SIGN signalling contributes to T FH differentiation. DCs were primed with lipopolysaccharide (LPS) and/or Lewis X (LeX), and cocultured with naive CD4 + T cells. After restimulation, we measured intracellular expression of T FH ‘master’ transcription factor Bcl-6 (ref. 14 ). T FH cells that induce GC formation and provide B-cell help in vivo are further characterized by high surface expression of receptors CXCR5 and PD-1, as well as secretion of IL-21 and low expression of transcription factor Foxp1, a negative regulator of IL-21 expression [2] , [3] , [17] , [21] , [22] , [23] , [24] . Strikingly, LPS/LeX-primed DCs induced strong expression of Bcl-6 in differentiated T H cells; we measured 12.0±3.9% ( n =11, P =0.0001, Student’s t -test) Bcl-6 + T H cells 24 h after restimulation ( Fig. 1a ). These in vitro generated Bcl-6 + T H cells also stained positive for CXCR5, while PD-1 expression was high and intracellular Foxp1 expression low ( Fig. 1b ), similar to in vivo generated T FH cells. Bcl-6 − cells were both negative and positive for CXCR5 expression, showed low-to-intermediate PD-1 and high Foxp1 expression ( Fig. 1c ), most likely representing T H 1 and T H 2 populations, with CXCR5 known to be expressed on T H 2 cells [21] . Induction of T FH cells was dependent on DC-SIGN signalling as DC priming in the presence of blocking DC-SIGN antibodies completely abrogated Bcl-6 + T H differentiation ( Fig. 1a,c ). Our naive T-cell pool contained no Bcl-6 + cells, indicating that DC-SIGN-primed DCs induced T H differentiation and not just proliferation. Neither immature DCs (iDCs), LeX-primed DCs nor LPS-primed DCs induced any Bcl-6-expressing T H cells ( Fig. 1a,c ). T FH differentiation was already optimal at 24 h after restimulation ( Fig. 1c ). We confirmed induction of Bcl-6 expression at the mRNA level in differentiated T H cells by LPS/LeX-primed DCs, but neither by iDCs nor by LPS-primed DCs, in a DC-SIGN-dependent manner ( Fig. 1d ). Bcl-6 activation in T FH cells is crucial for expression of IL-21, the main effector cytokine of T FH cells [13] , [14] , [15] . DC-SIGN-dependent T FH differentiation induced by DCs primed with LPS/LeX coincided with strong induction of IL-21 expression at both the mRNA and protein level, while LPS-primed DCs only induced minimal IL-21 expression by differentiated T H cells ( Fig. 1e,f ). IL-21 can also be secreted by T H -17 cells [25] ; however, neither LPS- nor LPS/LeX-primed DCs induced T H -17 differentiation as determined by mRNA expression of T H -17 ‘master’ regulator RORγt [25] ( Supplementary Fig. 1 ), confirming that T FH cells are the only source of IL-21 after T H differentiation by LPS/LeX-primed DCs. Thus, triggering of TLR4 and fucose-specific DC-SIGN signalling specifically primes DCs to induce Bcl-6 + CXCR5 + PD-1 hi Foxp1 lo T FH polarization. 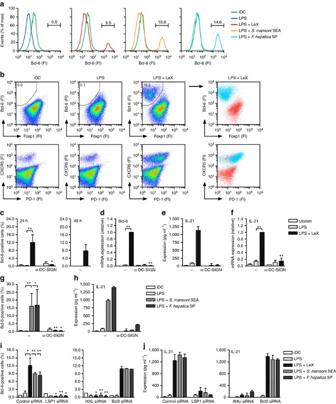Figure 1: DC-SIGN signalling by fucose-based PAMPs leads to IL-21-producing Bcl-6+TFHdevelopment. (a,c,g,i) THpolarization was determined by flow cytometry (FI, fluorescence intensity) 24 (a,g,i) or 48 (c) hours after restimulation by staining for intracellular Bcl-6 (TFH) expression after coculture of naive CD4+T cells with immature DCs (iDCs) or DCs primed with LPS plus LeX,S. mansonisoluble egg antigen (SEA) orF. hepaticasoluble products (SP), in the absence or presence of blocking DC-SIGN antibodies (c,g), or after LSP1, IKKε or Bcl3 silencing by RNA interference (siRNA) (i). Numbers above marker (a) indicate % Bcl-6+cells. **P<0.01, *P<0.05 (Student’st-test). (b) Bcl-6, CXCR5, PD-1 and Foxp1 expression was determined by flow cytometry 24 h after restimulation, after coculture of naive CD4+T cells with iDCs or DCs primed with LPS plus LeX. Numbers in gate indicate % Bcl-6+cells. Bcl-6+cells are represented in cyan and Bcl-6−cells in red in right panels. (d,f) Bcl-6 (d) and IL-21 (f) mRNA expression by differentiated T cells 24 h after restimulation, after coculture with iDCs or DCs primed with LPS plus LeX, in the absence or presence of blocking DC-SIGN antibodies, measured by real-time PCR, normalized to GAPDH and set at 1 in differentiated T cells cocultured with LPS/LeX-primed DCs. **P<0.01, *P<0.05 (Student’st-test). (e,h,j) IL-21 secretion in supernatants of differentiated T cells 24 h after restimulation, after coculture with iDCs or DCs primed with LPS plus LeX,S. mansoniSEA orF. hepaticaSP, in the absence or presence of blocking DC-SIGN antibodies (e,h), or after LSP1, IKKε or Bcl3 silencing (j) was measured by ELISA. Data are representative of at least eleven (a, LeX;c, 24 h without block), five (a, SEA and SP;g, 24 h without block), two (b), three (c,g, 24 h with block;c, 48 h;i,j), nine (d,f) or four (e,h) independent experiments (mean±s.d. inc,d,f,g,i; mean±s.d. of duplicates ine,h,j). Unstim, unstimulated. Figure 1: DC-SIGN signalling by fucose-based PAMPs leads to IL-21-producing Bcl-6 + T FH development. ( a , c , g , i ) T H polarization was determined by flow cytometry (FI, fluorescence intensity) 24 ( a , g , i ) or 48 ( c ) hours after restimulation by staining for intracellular Bcl-6 (T FH ) expression after coculture of naive CD4 + T cells with immature DCs (iDCs) or DCs primed with LPS plus LeX, S. mansoni soluble egg antigen (SEA) or F. hepatica soluble products (SP), in the absence or presence of blocking DC-SIGN antibodies ( c , g ), or after LSP1, IKKε or Bcl3 silencing by RNA interference (siRNA) ( i ). Numbers above marker ( a ) indicate % Bcl-6 + cells. ** P< 0.01, * P< 0.05 (Student’s t -test). ( b ) Bcl-6, CXCR5, PD-1 and Foxp1 expression was determined by flow cytometry 24 h after restimulation, after coculture of naive CD4 + T cells with iDCs or DCs primed with LPS plus LeX. Numbers in gate indicate % Bcl-6 + cells. Bcl-6 + cells are represented in cyan and Bcl-6 − cells in red in right panels. ( d , f ) Bcl-6 ( d ) and IL-21 ( f ) mRNA expression by differentiated T cells 24 h after restimulation, after coculture with iDCs or DCs primed with LPS plus LeX, in the absence or presence of blocking DC-SIGN antibodies, measured by real-time PCR, normalized to GAPDH and set at 1 in differentiated T cells cocultured with LPS/LeX-primed DCs. ** P< 0.01, * P< 0.05 (Student’s t -test). ( e , h , j ) IL-21 secretion in supernatants of differentiated T cells 24 h after restimulation, after coculture with iDCs or DCs primed with LPS plus LeX, S. mansoni SEA or F. hepatica SP, in the absence or presence of blocking DC-SIGN antibodies ( e , h ), or after LSP1, IKKε or Bcl3 silencing ( j ) was measured by ELISA. Data are representative of at least eleven ( a , LeX; c , 24 h without block), five ( a , SEA and SP; g , 24 h without block), two ( b ), three ( c , g , 24 h with block; c , 48 h; i , j ), nine ( d , f ) or four ( e , h ) independent experiments (mean±s.d. in c , d , f , g , i ; mean±s.d. of duplicates in e , h , j ). Unstim, unstimulated. Full size image We next investigated whether fucose-based PAMPs also induced T FH differentiation. Soluble egg antigen (SEA) derived from helminth Schistosoma mansoni express fucose-containing LeX and LDN-F structures, whereas adult Fasciola hepatica flatworms express LDN-F [26] that mediate interactions with DC-SIGN [27] ( Supplementary Fig. 2 ). DCs primed with LPS plus either S. mansoni SEA or F. hepatica soluble products (SP) also induced T FH differentiation as determined by percentages of Bcl-6 + cells and Bcl-6 mRNA expression ( Fig. 1a,f and Supplementary Fig. 3 ). Again, Bcl-6 + T H cells were further characterized as CXCR5 + , PD-1 hi and Foxp1 lo ( Supplementary Fig. 3 ). DCs primed with S. mansoni SEA or F. hepatica SP alone, similar to LeX alone, did not induce any T H proliferation. Moreover, DC priming with LPS plus either S. mansoni SEA or F. hepatica SP induced strong IL-21 secretion by differentiated T H cells, which was dependent on DC-SIGN signalling ( Fig. 1g and Supplementary Fig. 3 ), indicating that different fucose-based PAMPs can prime DCs via DC-SIGN to induce T FH polarization. We previously identified a fucose-specific DC-SIGN signalling pathway that primes TLR-stimulated DCs via LSP1-dependent IKKε-mediated Bcl3 activation to induce T H 2 responses [20] . We investigated whether this signalling pathway is similarly crucial for T FH differentiation. Both LSP1 and IKKε silencing in DCs by RNA interference ( Supplementary Fig. 4 ) inhibited T FH polarization by DCs primed with LPS plus either LeX, S. mansoni SEA or F. hepatica SP ( Fig. 1h,i ). Strikingly, T FH polarization by Bcl3-silenced LPS/LeX-primed DCs was unaffected and resulted in similar percentages of Bcl-6 + T FH cells and IL-21 production as compared with differentiation in response to control-silenced primed DCs ( Fig. 1h,i ). Thus, fucose engagement of DC-SIGN induces LSP1-IKKε-dependent but Bcl3-independent signalling that modulates TLR-induced priming of DCs, which is crucial for T FH polarization. Crosstalk between DC-SIGN and IFNR signalling activates ISGF3 To elucidate the mechanism behind DC-SIGN-IKKε-dependent priming of DCs for T FH differentiation, we considered different effectors of IKKε, besides CYLD [20] . Transcription factor STAT1 is a target for IKKε that induces phosphorylation at Ser708 (ref. 28 ). Ser708 phosphorylation of STAT1 is suggested to inhibit STAT1 homodimerization without disrupting STAT1–STAT2 dimerization [29] , which precedes recruitment of DNA binding unit IRF9 to form ISGF3 (ref. 30 ). Therefore, we investigated activation of STAT1 homodimers and ISGF3 after DC-SIGN triggering. We found that LPS stimulation of DCs induced nuclear translocation of STAT1 homodimers as determined by binding to IFN-γ-activated sites (GAS) [30] ( Fig. 2a ). Strikingly, LeX triggering of DC-SIGN largely inhibited LPS-induced STAT1–STAT1 binding to GAS sites ( Fig. 2a ), while strongly inducing ISGF3 formation, which bound to IFN-stimulated response elements (ISRE) [30] ( Fig. 2b ). Silencing of LSP1 or IKKε abrogated ISGF3 formation after DC-SIGN triggering ( Fig. 2d ) and led to induction of STAT1 homodimers ( Fig. 2c ). These data therefore indicate that DC-SIGN signalling via IKKε promotes ISGF3 formation, while inhibiting STAT1 homodimerization. 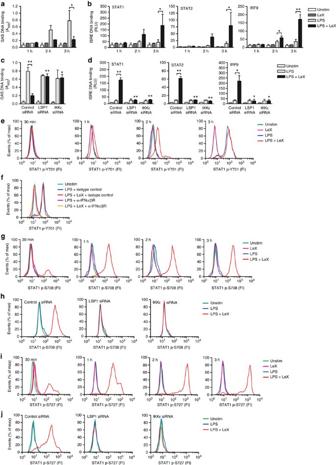Figure 2: Fucose-specific DC-SIGN signalling induces STAT1 phosphorylation at Ser708 and Ser727 via IKKε, thereby favouring ISGF3. (a–d) STAT1 homodimer and ISGF3 (STAT1–STAT2–IRF9 complex) activation in nuclear extracts of DCs 1, 2 or 3 (c,d) hours after stimulation with LPS and/or LeX, after LSP1 or IKKε silencing, measured by GAS (a,c) or ISRE (b,d) DNA binding ELISA, respectively. RLU, relative light units. **P<0.01, *P<0.05 (Student’st-test). (e–j) STAT1 phosphorylation at Tyr701 (e,f), Ser708 (g,h) or Ser727 (i,j) in DCs left unstimulated (Unstim; green) or 30 min, 1, 2 or 3 h (f,h,j) after stimulation with LPS (blue), LeX (pink) or LPS/LeX (red), in the presence of isotype control (LPS, purple; LPS/LeX, orange) or blocking IFNR antibodies (f) or after LSP1 or IKKε silencing (h,j), determined by flow cytometry (FI, fluorescence intensity). Data are representative of four (a,b,e,f,j), three (c,d,h) or five (g,i) independent experiments (mean±s.d. ina–d). Figure 2: Fucose-specific DC-SIGN signalling induces STAT1 phosphorylation at Ser708 and Ser727 via IKKε, thereby favouring ISGF3. ( a – d ) STAT1 homodimer and ISGF3 (STAT1–STAT2–IRF9 complex) activation in nuclear extracts of DCs 1, 2 or 3 ( c , d ) hours after stimulation with LPS and/or LeX, after LSP1 or IKKε silencing, measured by GAS ( a , c ) or ISRE ( b , d ) DNA binding ELISA, respectively. RLU, relative light units. ** P< 0.01, * P< 0.05 (Student’s t -test). ( e – j ) STAT1 phosphorylation at Tyr701 ( e , f ), Ser708 ( g , h ) or Ser727 ( i , j ) in DCs left unstimulated (Unstim; green) or 30 min, 1, 2 or 3 h ( f , h , j ) after stimulation with LPS (blue), LeX (pink) or LPS/LeX (red), in the presence of isotype control (LPS, purple; LPS/LeX, orange) or blocking IFNR antibodies ( f ) or after LSP1 or IKKε silencing ( h , j ), determined by flow cytometry (FI, fluorescence intensity). Data are representative of four ( a , b , e , f , j ), three ( c , d , h ) or five ( g , i ) independent experiments (mean±s.d. in a – d ). Full size image Formation of STAT1 homodimers as well as ISGF3 requires STAT1 phosphorylation at Tyr701, which controls dimerization of STAT1 with either STAT1 or STAT2, and is a prerequisite for nuclear translocation [30] , [31] . STAT1 phosphorylation at Tyr701 is driven by IFNR signalling and in the case of TLR triggering requires de novo synthesis of type I IFNs [30] , [32] . Indeed, TLR-induced IFNR-mediated STAT1 phosphorylation at Tyr701 was detected after 2 h and further increased after 3 h of stimulation ( Fig. 2e,f and Supplementary Fig. 5 ), which corresponded with GAS binding activity ( Fig. 2a,b ), and was not affected by DC-SIGN triggering. We next addressed whether DC-SIGN signalling directs the observed specific ISGF3 formation via STAT1 phosphorylation at Ser708. We detected efficient STAT1 phosphorylation at Ser708 after 30 min of stimulation with LPS/LeX ( Fig. 2g ), thus preceding IFNR-induced Tyr701 phosphorylation ( Fig. 2e ), whereas neither LPS nor LeX alone induced Ser708 phosphorylation ( Fig. 2g ). STAT1 Ser708 phosphorylation induced by LPS/LeX further increased over time ( Fig. 2g and Supplementary Fig. 5 ) in a LSP1- and IKKε-dependent manner ( Fig. 2h ). Notably, we also detected LSP1- and IKKε-dependent phosphorylation of STAT1 at Ser727 ( Fig. 2i,j and Supplementary Fig. 5 ), a site that resides in the transactivation domain of STAT1 and strongly enhances its transactivation potential [33] . Like Ser708 phosphorylation, IKKε-mediated Ser727 phosphorylation was irrespective of IFNR signalling ( Supplementary Fig. 5 ). These data indicate that DC-SIGN-IKKε-dependent signalling directs preferential formation of ISGF3 via STAT1 phosphorylation at Ser708, while enhancing ISGF3 transactivation activity via Ser727 phosphorylation. Both STAT1 homodimers and ISGF3 are involved in an autocrine positive feedback loop to boost type I IFN expression via induction of IFN-stimulated genes (ISGs) [34] . We next investigated whether DC-SIGN signalling enhanced type I IFN responses through ISGF3. LPS induced IFN-β mRNA expression early after 2 h as well as a second peak at 6 h post stimulation ( Fig. 3a ), which was dependent on IFNR signalling ( Fig. 3b ). LPS/LeX costimulation significantly enhanced and prolonged late IFN-β expression, which depended on DC-SIGN-induced IKKε activation and ISGF3 formation as determined by silencing of IKKε and IRF9, the DNA binding unit of ISGF3 ( Fig. 3a ). Transcription factor IRF7 is a known ISG as well as a regulator of IFN-β transcription [34] . DC-SIGN triggering significantly enhanced LPS-induced IFN-mediated IRF7 expression in an IKKε- and IRF9-dependent manner ( Fig. 3c,d ). Silencing of IRF7 abrogated the increased type I IFN responses, confirming that the DC-SIGN-mediated autocrine feedback loop on IFN-β expression was dependent on IRF7 expression ( Fig. 3a ). Expression of archetypical ISGs MxA and OAS1 (ref. 34 ) was also strongly enhanced after LPS/LeX costimulation ( Supplementary Fig. 6 ). These data show that crosstalk between fucose-specific DC-SIGN signalling and IFNR signalling specifically activates ISGF3, which might regulate a gene programme that underlies DC-SIGN-dependent T FH polarization by primed DCs. 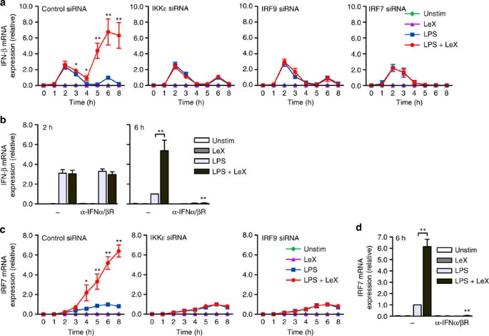Figure 3: Fucose-specific DC-SIGN signalling enhances type I IFN responses via ISGF3-dependent IRF7 expression. (a–d) IFN-β (a,b) and IRF7 (c,d) mRNA expression by DCs at indicated times after stimulation with LPS and/or LeX, after IKKε (a,c), IRF9 (a,c) or IRF7 (a) silencing, or in the absence or presence of blocking IFNR antibodies (b,d), measured by real-time PCR, normalized to GAPDH and set at 1 in 6 h LPS-stimulated cells. **P<0.01, *P<0.05 (Student’st-test). Data are representative of at least four (a,c) or five (b,d) independent experiments (mean±s.d.). Unstim, unstimulated. Figure 3: Fucose-specific DC-SIGN signalling enhances type I IFN responses via ISGF3-dependent IRF7 expression. ( a – d ) IFN-β ( a , b ) and IRF7 ( c , d ) mRNA expression by DCs at indicated times after stimulation with LPS and/or LeX, after IKKε ( a , c ), IRF9 ( a , c ) or IRF7 ( a ) silencing, or in the absence or presence of blocking IFNR antibodies ( b , d ), measured by real-time PCR, normalized to GAPDH and set at 1 in 6 h LPS-stimulated cells. ** P< 0.01, * P< 0.05 (Student’s t -test). Data are representative of at least four ( a , c ) or five ( b , d ) independent experiments (mean±s.d.). Unstim, unstimulated. Full size image Fucose-specific DC-SIGN signalling enhances IL-27 expression We next set out to find the factor(s) that orchestrate DC-SIGN-dependent priming of DCs for T FH differentiation. Type I IFN signalling in DCs has previously been reported to be involved in the development of T FH cells in mice via the induction of IL-6 (ref. 35 ). We have previously shown that IL-6 expression is downregulated in response to TLR4 and fucose-specific DC-SIGN costimulation via a DC-SIGN-induced IKKε-Bcl3 pathway [20] . Here we found that IL-6 expression in response to LPS/LeX stimulation was independent of IFNR triggering or ISGF3 activation, as determined by blocking IFNR antibodies and IRF9 silencing, respectively ( Fig. 4a and Supplementary Fig. 7 ), suggesting that IL-6 is not the crucial factor that underlies DC-SIGN-dependent T FH polarization by LPS/LeX-primed DCs. 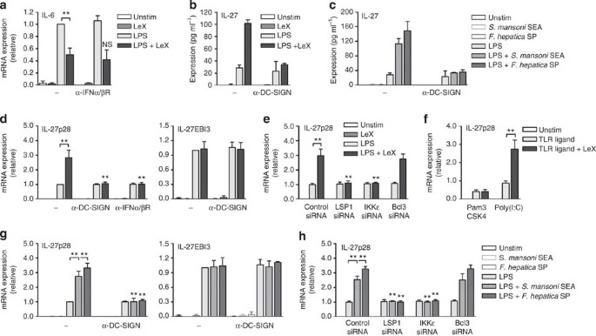Figure 4: Fucose-specific DC-SIGN signalling specifically upregulates IL-27p28 via IKKε. (a,d–h) IL-6 (a), IL-27p28 (d–h) and IL-27EBI3 (d,g) mRNA expression by DCs 6 hours after stimulation with LPS, PamCSK3 or poly(I:C) and/or LeX,S. mansoniSEA orF. hepaticaSP, in the absence or presence of blocking IFNR (a,d) or DC-SIGN (d,g) antibodies, or after LSP1, IKKε or Bcl3 silencing (e,g), measured by real-time PCR, normalized to GAPDH and set at 1 in TLR-stimulated cells. **P<0.01, NS, not significant (Student’st-test). (b,c) IL-27 secretion in supernatants of DCs 24 h after stimulation with LPS and/or LeX,S. mansoniSEA orF. hepaticaSP, in the absence or presence of blocking DC-SIGN antibodies. Data are representative of at least eight (a), four (b,c,g,h), five (d), nine (e) or seven (f) independent experiments (mean±s.d. ina,d–h; mean±s.d. of duplicates inb,c). Unstim, unstimulated. Figure 4: Fucose-specific DC-SIGN signalling specifically upregulates IL-27p28 via IKKε. ( a , d – h ) IL-6 ( a ), IL-27p28 ( d – h ) and IL-27EBI3 ( d , g ) mRNA expression by DCs 6 hours after stimulation with LPS, PamCSK3 or poly(I:C) and/or LeX, S. mansoni SEA or F. hepatica SP, in the absence or presence of blocking IFNR ( a , d ) or DC-SIGN ( d , g ) antibodies, or after LSP1, IKKε or Bcl3 silencing ( e , g ), measured by real-time PCR, normalized to GAPDH and set at 1 in TLR-stimulated cells. ** P< 0.01, NS, not significant (Student’s t -test). ( b , c ) IL-27 secretion in supernatants of DCs 24 h after stimulation with LPS and/or LeX, S. mansoni SEA or F. hepatica SP, in the absence or presence of blocking DC-SIGN antibodies. Data are representative of at least eight ( a ), four ( b , c , g , h ), five ( d ), nine ( e ) or seven ( f ) independent experiments (mean±s.d. in a , d – h ; mean±s.d. of duplicates in b , c ). Unstim, unstimulated. Full size image Since T FH generation is impaired in mice lacking IL-27R (ref. 36 ) and the promoter region of IL-27 , which encodes cytokine subunit IL-27p28, contains a functional ISRE [37] , we investigated IL-27 expression by DC-SIGN. Strikingly, LeX stimulation enhanced LPS-induced IL-27 expression by DCs several fold in a DC-SIGN-dependent manner ( Fig. 4b ). LeX, S. mansoni SEA and F. hepatica SP alone did not induce IL-27 ( Fig. 4b,c ). IL-27 is a heterodimeric cytokine composed of IL-27p28 and Epstein-Barr virus-induced gene 3 (EBI3) subunits [38] . We found that IL-27 protein expression was modulated by DC-SIGN signalling at the level of IL-27p28 transcription; while both IL-27p28 and IL-27EBI3 mRNA expression was induced by LPS alone, LeX costimulation enhanced IL-27p28 mRNA levels approximately threefold (2.6±0.27, n =10, P <0.001, Student’s t -test) in a DC-SIGN- and IFNR-dependent manner, whereas it did not affect EBI3 transcription ( Fig. 4d ). Furthermore, both LSP1 and IKKε silencing abrogated LeX-induced increase of IL-27p28 mRNA expression after LPS stimulation ( Fig. 4e ). In addition, LeX increased IL-27p28 mRNA expression after TLR3 stimulation with poly(I:C), but not after TLR2 triggering with Pam3CSK4 ( Fig. 4f ). This reflects the inability of TLR2 but not TLR3 to induce IFN-β synthesis ( Supplementary Fig. 8 ), which is required for crosstalk with DC-SIGN signalling to induce ISGF3 formation and as such for ISGF3-dependent IL-27p28 upregulation ( Fig. 4d ). Parasites such as S. mansoni carry or secrete TLR3 and TLR4 ligands [39] , [40] that makes IFNR- and DC-SIGN-driven ISGF3 formation during parasite infections physiologically relevant. Interfering with DC-SIGN signalling via blocking DC-SIGN antibodies, LSP1 or IKKε silencing completely abrogated IL-27p28 upregulation by parasitic PAMPs ( Fig. 4g,h ). As expected, Bcl3 silencing had no effect on LeX modulation of LPS-induced IL-27p28 mRNA expression ( Fig. 4e,h ). These data show that DC-SIGN triggering affects IL-27 expression via a LSP1- and IKKε-dependent increase in IL-27p28 expression. IKKε-dependent ISGF3 activation enhances IL-27 transcription To elucidate the role of ISGF3 in IL-27p28 expression in response to DC-SIGN signalling, we performed chromatin immunoprecipitation (ChIP) assays. We observed that both STAT1 and IRF9 were bound to the ISRE within the IL-27 promoter after LPS/LeX stimulation ( Fig. 5a ). To establish whether STAT1 binds as part of ISGF3 to the IL-27 ISRE, we performed re-ChIP experiments in which we performed a second immunoprecipitation with STAT2 or IRF9 antibodies on DNA–STAT1 complexes. We detected both STAT1–STAT2 and STAT1–IRF9 complexes bound to the IL-27 promoter after LPS/LeX stimulation ( Fig. 5b ). Silencing of IRF9 completely abrogated STAT1 recruitment to the IL-27 ISRE ( Fig. 5c ), indicating that all STAT1 bound to IL-27 is part of ISGF3 complexes. ISGF3 binding could already be detected 2 h post stimulation and further increased after 3 h of LPS/LeX stimulation ( Fig. 5c ), which follows the nuclear appearance of ISGF3 ( Fig. 2b ). Moreover, LSP1 and IKKε silencing abrogated binding of ISGF3 to IL-27 ( Fig. 5c ). These results show that DC-SIGN signalling via IKKε results in ISGF3 recruitment to the IL-27 promoter. 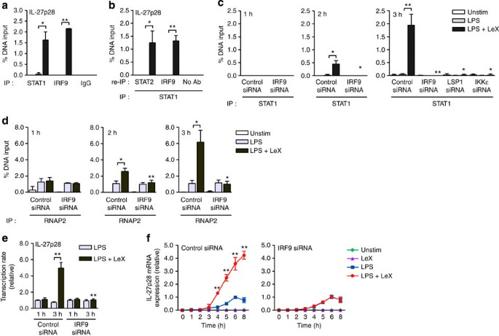Figure 5: IKKε-dependent ISGF3 activation acceleratesIL-27transcription via RNAP2 recruitment. (a–d) STAT1 (a,c), IRF9 (a), STAT1–STAT2 and STAT1–IRF9 (ISGF3;b) and RNA polymerase II (RNAP2) (d) recruitment to ISRE binding motif (a–c) and TATA box (d) of theIL-27promoter in DCs at indicated times (3 hours ina,b) after stimulation with LPS and/or LeX, after IRF9, LSP1 or IKKε silencing, determined by ChIP (a,c,d) and re-ChIP (b) assay. IgG and no antibody (Ab) indicate negative controls. Data are expressed as % input DNA. **P<0.01, *P<0.05 (Student’st-test). (e)IL-27transcription rate in DCs at indicated times after stimulation with LPS and/or LeX, after IRF9 silencing, determined by nuclear run-on assay, normalized to β-actin and set at 1 in 1 h LPS-stimulated control-silenced DCs. **P<0.01 (Student’st-test). (f) IL-27p28 mRNA expression by DCs over time after stimulation with LPS and/or LeX, after IRF9 silencing, measured by real-time PCR, normalized to GAPDH and set at 1 in 6 h LPS-stimulated cells. **P<0.01 (Student’st-test). Data are representative of at least four (a,e,f) or three (b–d) independent experiments (mean±s.d.). IP, immunoprecipitation; Unstim, unstimulated. Figure 5: IKKε-dependent ISGF3 activation accelerates IL-27 transcription via RNAP2 recruitment. ( a – d ) STAT1 ( a , c ), IRF9 ( a ), STAT1–STAT2 and STAT1–IRF9 (ISGF3; b ) and RNA polymerase II (RNAP2) ( d ) recruitment to ISRE binding motif ( a – c ) and TATA box ( d ) of the IL-27 promoter in DCs at indicated times (3 hours in a , b ) after stimulation with LPS and/or LeX, after IRF9, LSP1 or IKKε silencing, determined by ChIP ( a , c , d ) and re-ChIP ( b ) assay. IgG and no antibody (Ab) indicate negative controls. Data are expressed as % input DNA. ** P< 0.01, * P< 0.05 (Student’s t -test). ( e ) IL-27 transcription rate in DCs at indicated times after stimulation with LPS and/or LeX, after IRF9 silencing, determined by nuclear run-on assay, normalized to β-actin and set at 1 in 1 h LPS-stimulated control-silenced DCs. ** P< 0.01 (Student’s t -test). ( f ) IL-27p28 mRNA expression by DCs over time after stimulation with LPS and/or LeX, after IRF9 silencing, measured by real-time PCR, normalized to GAPDH and set at 1 in 6 h LPS-stimulated cells. ** P< 0.01 (Student’s t -test). Data are representative of at least four ( a , e , f ) or three ( b – d ) independent experiments (mean±s.d.). IP, immunoprecipitation; Unstim, unstimulated. Full size image Recent studies have demonstrated that ISGF3 recruits RNAP2 to ISRE-responsive promoters [41] . Further ChIP analyses showed that LPS induced low levels of RNAP2 recruitment to IL-27 , which was strongly enhanced by LeX ( Fig. 5d ). This increase in recruitment of RNAP2 followed ISGF3 binding to the IL-27 promoter in time and was completely abolished by IRF9 silencing ( Fig. 5d ). These data strongly indicate that DC-SIGN signalling increases transcriptional induction of IL-27 via ISGF3-facilitated recruitment of RNAP2. Therefore, we determined the effect of DC-SIGN on the transcription rate from the IL-27 gene at different time points. After 1 h of stimulation, we detected similar IL-27 transcription rates in LPS- and LPS/LeX-stimulated DCs ( Fig. 5e ). However, 3 h post stimulation, LeX enhanced the LPS-induced IL-27 transcription rate approximately fivefold (4.97±0.68, n =4, P =0.001, Student’s t -test; Fig. 5e ). IRF9 silencing completely abrogated this increase in transcription rate ( Fig. 5e ), demonstrating that ISGF3 activation is instrumental in DC-SIGN-induced upregulation of IL-27p28 expression via RNAP2 recruitment to the IL-27 promoter. While LPS-induced expression of IL-27p28 showed transient mRNA accumulation that peaked at 6 h post stimulation, LPS/LeX stimulation significantly accelerated IL-27 transcription from 3 h post stimulation, which further increased over time ( Fig. 5f ). IRF9 silencing completely blocked any increase in IL-27 transcription in response to LeX ( Fig. 5f ), supporting our conclusion that ISGF3 activation is required for enhancement of IL-27 expression by DC-SIGN triggering via RNAP2 recruitment. DC-SIGN-induced IL-27 expression directs T FH polarization To elucidate the contribution of DC-SIGN-induced IL-27 to T FH polarization after DC priming, we neutralized IL-27-mediated effects in T H differentiation assays during DC-T-cell coculture. Remarkably, neutralizing IL-27 antibodies completely abrogated T FH polarization by LPS plus fucose-primed DCs ( Fig. 6a–c ). Similarly, induction of T FH cells and IL-21 secretion by differentiated T H cells in response to DCs primed with LPS plus S. mansoni SEA or F. hepatica SP was completely blocked by neutralizing IL-27 antibodies ( Fig. 6a–c ). Neutralizing IL-27 antibodies did not affect DC-SIGN-dependent T H 2 polarization by LPS/LeX-primed DCs ( Supplementary Fig. 9 ). Vice versa, the addition of rhIL-27 to T cells cocultured with LPS-primed DCs induced T FH polarization in the absence of LeX priming of DCs, indicating that a threshold level of IL-27—as induced after DC-SIGN triggering—is required for T FH induction ( Fig. 6d,e ). In contrast, addition of rhIL-6 did not affect T FH differentiation in response to LPS-primed DCs ( Fig. 6d,e ). Neutralizing IL-6 antibodies did partially block T FH polarization in response to LPS/LeX-primed DCs ( Fig. 6d,e ). These results indicate that both IL-27 and IL-6 are required, but DC-SIGN-induced IL-27 provides the decisive signal for T FH polarization. Moreover, blocking DC-SIGN-mediated ISGF3 activation and hence IL-27 expression via IRF9 silencing in DCs, similarly as neutralizing IL-27 antibodies, blocked Bcl-6 induction in and IL-21 secretion by differentiated T H cells in response to LPS plus fucose-primed DCs ( Fig. 6f,g ), without affecting T H 2 polarization ( Supplementary Fig. 9 ). Thus, DC-SIGN-induced expression of IL-27 is crucial to priming DCs for T FH polarization. 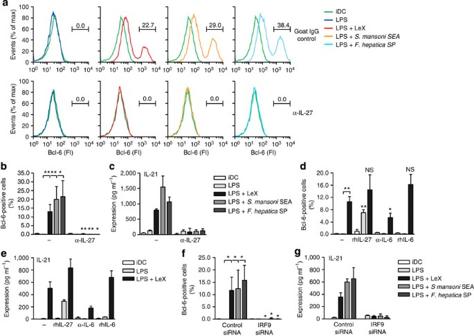Figure 6: DC-SIGN-induced IL-27 expression is crucial for TFHpolarization. (a,b,d,f) THpolarization was determined by flow cytometry (FI, fluorescence intensity), 24 hours after restimulation, by staining for intracellular Bcl-6 (TFH) expression after coculture of naive CD4+T cells with immature DCs (iDC) or DCs primed with LPS plus LeX,S. mansoniSEA orF. hepaticaSP. IL-27 (a,b,f) or IL-6 (d) stimulation of T cells was inhibited by neutralizing IL-27 (a,b) or IL-6 (d) antibodies during DC-T-cell coculture, with normal goat IgG as control (a), or via IRF9 silencing of DCs (f). Ind, DC-T cocultures were supplemented with rhIL-27 or rhIL-6. Numbers above marker (a) indicate % Bcl-6+cells. **P<0.01, *P<0.05, NS=not significant (Student’st-test). (c,e,g) IL-21 secretion in supernatants of differentiated T cells 24 h after restimulation, after coculture with iDCs or DCs primed with LPS plus LeX,S. mansoniSEA orF. hepaticaSP, measured by ELISA. IL-27 and IL-6 effects on T cells were either blocked or stimulated as described above. Data are representative of nine (a,c, LeX), five (a,c, SEA, SP), eight (b) or four (d–g) independent experiments (mean±s.d. inb,d,f; mean±s.d. of duplicates inc,e,g). Figure 6: DC-SIGN-induced IL-27 expression is crucial for T FH polarization. ( a , b , d , f ) T H polarization was determined by flow cytometry (FI, fluorescence intensity), 24 hours after restimulation, by staining for intracellular Bcl-6 (T FH ) expression after coculture of naive CD4 + T cells with immature DCs (iDC) or DCs primed with LPS plus LeX, S. mansoni SEA or F. hepatica SP. IL-27 ( a , b , f ) or IL-6 ( d ) stimulation of T cells was inhibited by neutralizing IL-27 ( a , b ) or IL-6 ( d ) antibodies during DC-T-cell coculture, with normal goat IgG as control ( a ), or via IRF9 silencing of DCs ( f ). In d , DC-T cocultures were supplemented with rhIL-27 or rhIL-6. Numbers above marker ( a ) indicate % Bcl-6 + cells. ** P< 0.01, * P< 0.05, NS=not significant (Student’s t -test). ( c , e , g ) IL-21 secretion in supernatants of differentiated T cells 24 h after restimulation, after coculture with iDCs or DCs primed with LPS plus LeX, S. mansoni SEA or F. hepatica SP, measured by ELISA. IL-27 and IL-6 effects on T cells were either blocked or stimulated as described above. Data are representative of nine ( a , c , LeX), five ( a , c , SEA, SP), eight ( b ) or four ( d – g ) independent experiments (mean±s.d. in b , d , f ; mean±s.d. of duplicates in c , e , g ). Full size image T FH cells promote B-cell IgG production and survival T FH cells provide cognate help to B cells to ensure long-lived humoural immunity after infection [2] , [3] . We performed B-cell help assays to establish whether T FH polarization via IL-27 in response to fucose-specific DC-SIGN-mediated priming of DCs induces antibody production by B cells. We isolated CD19 + B cells from peripheral blood containing both IgM-producing naive B cells and isotype-committed memory B cells. Next, we cocultured these B cells with T H cells differentiated by differently primed DCs and after T-cell-specific restimulation, we measured IgM and IgG production by activated B cells. T H cells differentiated by LPS-primed DCs induced production of both IgM and IgG by B cells ( Fig. 7 ). However, IgG production was strongly induced and IgM production decreased after coculture of B cells with DCs primed with LPS plus fucose-based PAMPs ( Fig. 7 ). Strikingly, blocking DC-SIGN-mediated T H differentiation via neutralizing IL-27 antibodies during DC-T-cell coculture strongly diminished IgG production by activated B cells while leaving IgM production undisturbed ( Fig. 7a ). T FH cells also promote B-cell survival in GCs via PD-1 signalling [42] . Annexin V/propidium iodide (PI) stainings showed that T FH cells generated in vitro by DCs primed with fucose PAMPs also supported B-cell survival, in an IL-27-dependent manner ( Fig. 7b ). These results suggest that fucose-specific DC-SIGN-mediated priming of DCs is essential to the induction of T FH cells and cognate B-cell help to induce IgG production. 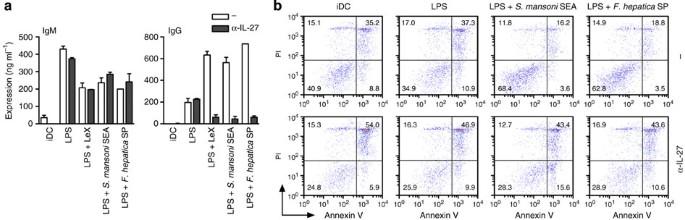Figure 7: DC-SIGN-induced IL-27 expression is crucial for B cells IgG production via T-cell help. (a) IgM and IgG secretion in supernatants of B cells 7 days after stimulation with T cells that were differentiated after coculture with immature DCs (iDCs) or DCs primed with LPS plus LeX,S. mansoniSEA orF. hepaticaSP, measured by ELISA. IL-27 effects on T cells were blocked by neutralizing IL-27 antibodies during DC-T-cell coculture. (b) B-cell survival 48 hours after stimulation with T cells that were differentiated after coculture with iDCs or DCs primed with LPS plusS. mansoniSEA orF. hepaticaSP was determined by flow cytometry via Annexin V-FITC/PI staining. Numbers in quadrants indicate % cells in each. Data are representative of three (a) or two (b) independent experiments (mean±s.d. of duplicates ina). Figure 7: DC-SIGN-induced IL-27 expression is crucial for B cells IgG production via T-cell help. ( a ) IgM and IgG secretion in supernatants of B cells 7 days after stimulation with T cells that were differentiated after coculture with immature DCs (iDCs) or DCs primed with LPS plus LeX, S. mansoni SEA or F. hepatica SP, measured by ELISA. IL-27 effects on T cells were blocked by neutralizing IL-27 antibodies during DC-T-cell coculture. ( b ) B-cell survival 48 hours after stimulation with T cells that were differentiated after coculture with iDCs or DCs primed with LPS plus S. mansoni SEA or F. hepatica SP was determined by flow cytometry via Annexin V-FITC/PI staining. Numbers in quadrants indicate % cells in each. Data are representative of three ( a ) or two ( b ) independent experiments (mean±s.d. of duplicates in a ). Full size image Induction of T FH cells is essential for antibody-mediated immunity via GC formation and differentiation of memory B cells and plasma cells. Here we demonstrate that engagement of DC-SIGN by fucose-based PAMPs primes DCs for T FH polarization. At the molecular level, we identified IKKε as the crucial conductor for T FH differentiation ( Supplementary Fig. 10 ). Crosstalk between fucose-specific DC-SIGN and type I IFNR signalling favoured formation of ISGF3 complexes consisting of STAT1–STAT2 and IRF9 over STAT1 homodimerization owing to IKKε-mediated STAT1 phosphorylation at Ser708. ISGF3 increased the transcription rate of the IL-27 gene, encoding the IL-27p28 subunit, by recruiting RNAP2 to its promoter. We found that the increase in IL-27 production was crucial for the development of T FH cells and T-cell help to B cells for the production of IgG and survival, which might contribute to development of long-term humoural responses to, for example, parasites such as S. mansoni and F. hepatica that express various fucose-based glycan PAMPs [26] . The origin of T FH cells and their relationship with other T H subsets is the subject of ongoing investigations. New insights have led to a multistage, multifactorial model in which DCs initially prime T FH differentiation; however, these signals are thought to be transient, and B cells are required at a second stage to sustain T FH differentiation. In the absence of this second stage, T cells might revert and follow a different differentiation path depending on their unique microenvironments [2] , [43] . Our data show that fucose-primed DCs indeed induce T FH differentiation from naive T cells. Our data also suggest that T FH fate is established at the time of DC priming and develops exclusively of other T H subsets that opposes observations in mice immunized with S. mansoni SEA, where T FH cells seemed to convert from T H 2 precursor cells [44] ; we observed that generation of T FH and T H 2 subsets required different priming signals, as Bcl3 silencing in DCs did not affect T FH differentiation, while IRF9 silencing or neutralization of IL-27 signals did not interfere with T H 2 differentiation. We established the noncanonical kinase IKKε as the central player in T H polarization via DC-SIGN. IKKε is mostly known for its role in RIG-I-like receptor-mediated antiviral immunity via IRF3 and IRF7 phosphorylation to induce type I IFN production [45] . We have previously shown that IKKε recruitment to DC-SIGN in response to fucose binding leads to Bcl3-dependent priming of DCs for T H 2 polarization [20] . Here we demonstrated that IKKε also induced ISGF3-dependent T FH differentiation in response to fucose-based PAMPs. The induction of both T FH and T H 2 differentiation is required for production of high-affinity, class-switched antibodies and protective long-term humoural immunity [1] , [2] . IL-21 acts as a switch factor for human IgG1 and IgG3 (ref. 46 ). We show here that fucose priming of DCs induces differentiation of T FH cells that functionally instruct B cells in vitro to induce IgG production. Sequential switching of IgG cells to IgE is essential for the development of long-lived high-affinity IgE + plasma cells, for which T H 2-produced IL-4 acts as a switch factor [4] , [5] , [6] , [8] . Thus, our results suggest that DC-SIGN-mediated DC priming via IKKε can provide the signals for establishing long-term humoural immunity via induction of both T FH and T H 2. The role of IKKε in T FH differentiation revealed another level of crosstalk between innate signalling pathways. Here we demonstrated that crosstalk between IFNR and DC-SIGN signalling via IKKε is a prerequisite for T FH differentiation. IKKε induced STAT1 phosphorylation at Ser708 that favours the formation of ISGF3 complexes by interfering with STAT1 homodimerization, hence increasing IL-27 production and inducing T FH generation. IKKε phosphorylation of STAT2 in addition to STAT1 might further influence ISGF3 assembly [29] . However, although IKKε-mediated serine phosphorylation of STAT1 precedes TLR4-induced IFNR signalling, IFNR signalling is required for STAT1 phosphorylation at Tyr701 to induce heterodimerization between STAT1 and STAT2 (for ISGF3 formation) and STAT1 homodimerization [30] , [31] . A previous report suggested that phosphorylation of Ser708 and Tyr701 are mutually exclusive when Tyr701 phosphorylation preceded Ser708 phosphorylation [47] ; however, during costimulatory TLR4-DC-SIGN triggering, Ser708 phosphorylation exhibits faster kinetics than Tyr701 phosphorylation. Thus, de novo type I IFN synthesis induced by TLR signalling intersects with IKKε signalling to generate ISGF3 complexes. IFNR signalling alone cannot replace TLR signalling as MK2 activation is required for LSP1 phosphorylation and subsequent IKKε activation after DC-SIGN triggering. ISGF3 mediates its actions via ISRE sites and recruits RNAP2 to its target promoters, most likely via STAT2 within the ISGF3 complex [41] . Besides favouring ISGF3 formation via Ser708 phosphorylation, we also observed simultaneous Ser727 phosphorylation in an IKKε-dependent manner. Although Ser727 was not identified as a target for IKKε in mouse STAT1 (refs 28 , 29 ), we now show that IKKε is involved in Ser727 phosphorylation of human STAT1. Ser727 is present within the transactivation domain of STAT1, enhancing its transactivational activity [33] . Our results demonstrate that ISGF3 formation is not only dependent on DC-SIGN triggering but also implicate that ISGF3 activity is further boosted by IKKε-dependent DC-SIGN signalling. Type I IFN signalling in DCs has previously been reported to be involved in the development of T FH cells in mice via the induction of IL-6 (ref. 35 ). Our data show that in human DCs, IL-6 is a prerequisite but not sufficient for T FH induction, while its induction via TLR4 is independent of IFNR triggering. Here we show that IFNR- and IKKε-dependent ISGF3 formation induces IL-27, which is the decisive cytokine for T FH induction. The IL-27 promoter contains a ISRE binding site that can be sequentially bound by IRF1 or IRF3 and ISGF3 (ref. 37 ). We observed initial transcriptional activation of IL-27 due to TLR signalling before DC-SIGN-IKKε-induced ISGF3 activation, which was strongly accelerated once ISGF3 was bound and enhanced RNAP2 recruitment. IL-27 most likely acts in concert with other factors at the time of DC priming to induce T FH differentiation, such as IL-21 and IL-6 (refs 12 , 16 ). IL-27R deficiency also impairs T FH induction [36] . IL-27, IL-21 and IL-6 all have in common that they induce STAT3 activation, implying that STAT3-mediated signalling routes in T cells are important for T FH development [48] . Our data suggest a model in which threshold levels of IL-27 and IL-6 expression by DCs are required for efficient T FH differentiation. LPS-stimulated DCs produced substantial IL-6 (ref. 20 ), but low amounts of IL-27, that was insufficient for T FH differentiation. However, fucose-specific DC-SIGN signalling combined with LPS stimulation decreased IL-6 while enhancing IL-27 secretion, consequently inducing T FH development. Parasites such as S. mansoni carry or secrete TLR3 and TLR4 ligands [39] , [40] , underlining the physiological relevance of IFNR- and DC-SIGN-driven IL-27 expression during parasite infections. Thus, we have identified the molecular mechanisms behind fucose-specific triggering of DC-SIGN signalling that leads to increased IL-27 expression by LPS-stimulated DCs, which triggers a threshold for differentiation of T FH cells, which in turn induces specific IgG production by B cells. Unravelling the molecular requirements underlying DC-SIGN-mediated T FH development will help to identify potentials targets for effective vaccination strategies as well as treatment of immunological diseases that are characterized by insufficient or excessive antibody responses. Stimulation and RNA interference of DCs Peripheral blood mononuclear cells were isolated from buffy coats of healthy volunteer blood donors (Sanquin) by a Lymphoprep (Axis-Shield) gradient step, and monocytes were subsequently isolated by a Percoll (Amersham) gradient step. Monocytes were differentiated into iDCs in the presence of 500 U ml −1 IL-4 and 800 U ml −1 granulocyte-macrophage colony-stimulating factor (GM-CSF) (both Invitrogen), and used at day 6 or 7. This study was approved by the Medical Ethics Review Committee of the Academic Medical Center (AMC). DCs were stimulated with 10 ng ml −1 Salmonella typhosa LPS (Sigma), 10 μg ml −1 Pam3CSK4, 10 μg ml −1 poly(I:C) (both from Invivogen), 10 μg ml −1 Lewis X-PAA (Lectinity), 40 μg ml −1 SEA prepared from S. mansoni eggs (provided by F. Lewis, Biomedical Research Institute, Rockville, MD) or 40 μg ml −1 SPs prepared from adult F. hepatica worms (provided by L. Tielens, Utrecht University, The Netherlands). SEAs and SPs were prepared by homogenization of eggs or worms in 10 volumes of Tris–HCl (pH 8.0) via four times 30 s polytron pulses on ice, followed by four times 1 min sonication (21 kHz, with 7 μm amplitude) on ice. After centrifugation (10,000 g at 4 °C for 30 min), supernatants were filtered (0.45 μm) and stored at −80 °C (ref. 49 ). DCs were preincubated for 2 h with the following blocking antibodies: 20 μg ml −1 anti-DC-SIGN (AZN-D1; generated ‘in-house’ [50] ), 20 μg ml −1 anti-IFNα/βR2 (MMHAR-2; PBL Interferon Source) or 20 μg ml −1 mouse IgG2a isotype control antibodies (14-4724-85; eBioscience). DCs were transfected with 25 nM short interfering RNA (siRNA) using transfection reagents DF4 (Dharmacon) according to the manufacturer’s instructions. SMARTpool siRNAs used were as follows: LSP1 (M-012640-00), IKKε (M-003723-02), Bcl3 (M-003874-02), IRF9 (M-020858-02), IRF7 (M-011810-02) and non-targeting siRNA (D-001206-13) as a control (Dharmacon). Silencing of expression was verified by real-time PCR and flow cytometry; cell survival was determined by flow cytometry via Annexin V-fluorescein isothiocyanate (FITC)/PI staining (eBioscience) ( Supplementary Fig. 4 ). T-cell differentiation and B-cell help assay Naive CD4 + T cells were isolated from buffy coats of healthy blood donors (Sanquin) with human CD4 + T-cell isolation kit II (Miltenyi) by negative selection combined with depletion of CD45RO + memory T cells by staining with phycoerythrin (PE)-conjugated anti-CD45RO (80 μg ml −1 ; R0843; Dako), coated on anti-PE beads (Miltenyi). B cells were isolated from buffy coats of healthy blood donors (Sanquin) with human B-cell isolation kit II (Miltenyi) by negative selection; 95% of isolated cells were CD19 + , whereas 16% were IgD + CD27 − naive cells as determined by staining with anti-CD19 (1:25; HIB19; eBioscience), anti-IgD (1:20; IA6-2; Pharmingen) and anti-CD27 (1:20; LT27; eBioscience). This study was approved by the Medical Ethics Review Committee of the AMC. DCs were either silenced for indicated proteins or preincubated for 2 h with blocking DC-SIGN antibodies and activated for 48 h as indicated. IDCs were cultured in the presence of 1 μg ml −1 GM-CSF (Invitrogen). DCs were cocultured with naive CD4 + T cells (20,000 T cells/5,000 DCs) in the presence of 10 pg ml −1 Staphylococcus aureus enterotoxin B (Sigma). An amount of 30 ng ml −1 rhIL-27, 40 ng ml −1 rhIL-6 (both R&D Systems) or 5 μg ml −1 neutralizing antibodies against IL-27 (AF2526; R&D Systems), IL-6 (AF-206-NA; R&D Systems) or normal goat IgG (AB-108-C; R&D Systems), as a control, were added at this point. After 5 days, cells were further cultured with 10 U ml −1 IL-2 (Chiron). Resting T cells were restimulated after 12–16 days with 100 ng ml −1 PMA (Sigma) and 1 μg ml −1 ionomycin (Sigma). For flow cytometry analysis of differentiated T H cells, cells were first fixed at 24 or 48 h after restimulation in 3% para -formaldehyde for 10 min and permeabilized in 90% methanol at 4 °C for 16 h. Cells were stained with Alexa Fluor 647-conjugated anti-CXCR5 (1:20; 558113; BD Pharmingen), PerCP-Cy5.5-conjugated anti-PD-1 (1:20; 561273; BD Pharmingen), Alexa Fluor 488-conjugated anti-Foxp1 (1:20; IC45341G; R&D Systems) and anti-Bcl-6 (1:20; ab19011; Abcam), followed by incubation with PE-conjugated anti-rabbit (1:200; 711-116-152, Jackson ImmunoResearch). Analyses were performed on a FACS Canto (BD Biosciences). Supernatants of T cells were harvested 24 h after restimulation for IL-21 expression analysis by enzyme-linked immunosorbent assay (ELISA), while mRNA was isolated as described below for quantitative real-time PCR analysis of T H markers. For flow cytometry analysis of intracellular IL-4 (T H 2 cells) and IFN-γ (T H 1 cells) expression, cells were restimulated for 6 h, the last 4 h in the presence of 10 μg ml −1 brefeldin A (Sigma). Cells were stained with APC-conjugated anti-IL-4 (1:25; MP4-25D2; BD Biosciences) and FITC-conjugated anti-IFN-γ (1:5; 25723.11; BD Biosciences). DCs primed with 10 ng ml −1 LPS plus 1,000 U ml −1 IFN-γ (U-CyTech) or 1 μM PGE 2 (Sigma) were used as positive controls for T H 1 and T H 2 differentiation, respectively. For analysis of T-cell-dependent help to B cells for Ig production, resting differentiated T cells were cocultured with B cells (100,000 T cells/50,000 B cells) and restimulated with 1 μg ml −1 anti-CD3 (1XE; Sanquin) and 1 μg ml −1 anti-CD28 (15E8; Sanquin). B-cell survival was examined after 2 days by flow cytometry via Annexin V-FITC/PI staining (eBioscience). B cells were identified by staining with anti-CD19-APC (1:40; 345791; BD Biosciences). Supernatants were harvested after 7 days for analysis of B-cell IgM and IgG production by ELISA. DC-SIGN binding DC-SIGN binding of parasitic PAMPs was determined by DC-SIGN-Fc ELISA as described in ref. 50 . Cytokine and Ig production DC, T- or B-cell culture supernatants were harvested, and IL-21 (88-7216-22; eBioscience), IL-27 (88-7278-22; eBioscience), IgM (88-50620-22; eBioscience) and total IgG (88-50550-22; eBioscience) were measured by ELISA. Quantitative real-time PCR mRNA isolation, cDNA synthesis and PCR amplification in the presence of SYBR green in an ABI 7500 Fast PCR detection system (Applied Biosystems) were performed as described in ref. 20 . Specific primers were designed using Primer Express 2.0 (Applied Biosystems; Supplementary Table 1 ). The relative mRNA expression was obtained by setting N t (=2 Ct(GAPDH)−Ct(target) ) at 1 in TLR ligand-stimulated DCs or T cells primed with LPS- (RORγt) or LPS/LeX- (Bcl-6 and IL-21) stimulated DCs, within one experiment and for each donor. STAT1 and ISGF3 DNA binding Nuclear extracts of DCs were prepared using NucBuster protein extraction kit (Novagen). STAT1 GAS DNA binding was determined using TransAM STAT family kit (Active Motif). ISGF3 ISRE DNA binding was determined using Universal EZ-TFA Chemiluminescent Transcription Factor Assay (Millipore) in combination with 5′-biotin-labelled sense strand oligonucleotide 5′- CTCTGCAAGGGTCATCGGGGAAGCCTTTTCAAGGAAACGAAAGTGAACTC -3′ and unlabelled antisense strand 5′- GAGTTCACTTTCGTTTCCTTGAAAAGGCTTCCCCGATGACCCTTGCAGAG -3′. Bound ISGF3 was detected with anti-STAT1 (1:500; 9172; Cell Signaling), anti-STAT2 (1:100; 4594; Cell Signaling) and anti-IRF9 (1:500; sc-496X; Santa Cruz Biotechnology), followed by incubation with horseradish peroxidase (HRP)-conjugated anti-rabbit Ig (1:500; in kit) and chemiluminescence detection with a Synergy HT reader (Biotek). STAT1 phosphorylation Cells were first fixed in 3% para -formaldehyde for 10 min and permeabilized in 90% methanol at 4 °C for 30 min. Primary antibody incubation with anti-STAT1 p-S708 (ref. 47 ; 1:200; provided by M. Gale, Jr, University of Washington School of Medicine, Seattle, WA) and anti-STAT1 p-S727 (1:100; 9177; Cell Signaling) was followed by incubation with PE-conjugated anti-rabbit (1:200; 711-116-152, Jackson ImmunoResearch). STAT1 phosphorylation at Tyr701 was determined by direct labelling with Alexa Fluor 488-conjugated anti-STAT1 p-Y701 (1:1.67; 612596; BD Biosciences). Phosphorylation was analysed on a FACS Calibur (BD Biosciences). STAT1 phosphorylation was further determined in whole-cell extracts that were prepared using RIPA buffer (Cell Signaling). Proteins were resolved by SDS–polyacrylamide gel electrophoresis and detected by immunoblotting with anti-STAT1 p-S708 (1:250), anti-STAT1 p-S727 (1:1,000), anti-STAT1 p-Y701 (1:50) and anti-total STAT1 (1:1,000; 9172; Cell Signaling), followed by incubation with HRP-conjugated secondary antibody (1:2,500; 21230; Pierce) and ECL detection (Pierce). ChIP assay ChIP and re-ChIP assays were performed using ChIP-IT Express Enzymatic Shearing and ChIP-IT Express HT kits (both from Active Motif). Briefly, cells were fixed with 1% (vol/vol) para -formaldehyde, nuclei were isolated and chromatin DNA fragmented by enzymatic shearing (10 min, 37 °C). Protein–DNA complexes were immunoprecipitated using 4 μg anti-STAT1 (9172; Cell Signaling), anti-IRF9 (sc-496X; Santa Cruz), anti-RNAP2 (39097; Active Motif) or negative control IgG (sc-2027; Santa Cruz), and protein G-coated magnetic beads. For re-ChIP analyses, STAT1–DNA complexes were eluted from beads and desalted using the re-ChIP-IT kit (Active Motif). A second round of immunoprecipitation was performed with 4 μg anti-IRF9 or anti-STAT2 (39060; Active Motif). DNA was purified after reversal of crosslinks. Real-time PCR was performed with a primer set spanning both ISRE and TATA box of the IL-27 promoter ( Supplementary Table 1 ). Negative Control Primer Set 1 (Active Motif) was used as a negative control. To normalize for DNA input, a sample for each condition was taken along which had not undergone immunoprecipitation (‘input DNA’); results are expressed as % input DNA. Nuclear run-on assay Nuclei were isolated from DCs as described previously [51] . Transcription was allowed to proceed in the presence of 1 mM 16-biotin-UTP (Roche) at 26 °C for 20 min. Newly synthesized biotin-containing RNA was isolated with mRNA capture kit (Roche). cDNA synthesis and PCR amplification were performed as described above, except that expression was normalized using β-actin. The relative mRNA expression was obtained by setting N t at 1 in 1 h LPS-stimulated control-silenced DCs, within one experiment and for each donor. Statistical analysis Statistical analyses were performed using the Student’s t -test for paired observations. Statistical significance was set at P <0.05. How to cite this article: Gringhuis, S. I. et al . Fucose-based PAMPs prime dendritic cells for follicular T helper cell polarization via DC-SIGN-dependent IL-27 production. Nat. Commun. 5:5074 doi: 10.1038/ncomms6074 (2014).